Reductive cyanation of organic chlorides using CO2and NH3via Triphos–Ni(I) species Cyano-containing compounds constitute important pharmaceuticals, agrochemicals and organic materials. Traditional cyanation methods often rely on the use of toxic metal cyanides which have serious disposal, storage and transportation issues. Therefore, there is an increasing need to develop general and efficient catalytic methods for cyanide-free production of nitriles. Here we report the reductive cyanation of organic chlorides using CO 2 /NH 3 as the electrophilic CN source. The use of tridentate phosphine ligand Triphos allows for the nickel-catalyzed cyanation of a broad array of aryl and aliphatic chlorides to produce the desired nitrile products in good yields, and with excellent functional group tolerance. Cheap and bench-stable urea was also shown as suitable CN source, suggesting promising application potential. Mechanistic studies imply that Triphos-Ni(I) species are responsible for the reductive C-C coupling approach involving isocyanate intermediates. This method expands the application potential of reductive cyanation in the synthesis of functionalized nitrile compounds under cyanide-free conditions, which is valuable for safe synthesis of (isotope-labeled) drugs. Nitriles are key intermediates in production of pharmaceuticals, agrochemicals, organic materials, and functional materials [1] , [2] . Moreover, nitrile group serves as a versatile motif for the synthesis of aldehydes, ketones, carboxylic acids, alcohols, amides, amines, and heterocycles [3] . Significant progress has been made in transition-metal-catalyzed cyanation in the past century, among which cyanation of aryl (pseudo)halides is the most commonly used approach for selective synthesis of aryl nitriles [4] , [5] , [6] , [7] . Careful selection of cyanating reagents is usually required. In this regard, the direct use of metal/silyl cyanides or the in situ generation of cyanide ion is often involved (Fig. 1a, b : K 4 [Fe(CN) 6 ] [8] , [9] , [10] , [11] , [12] , [13] , [14] , K 3 [Fe(CN) 6 ] [15] , ethyl cyanoacetate [16] , [17] , acetone cyanohydrin [18] , [19] , [20] , butyronitrile [21] , 4-cyanopyridine N -oxide [22] , formamide [23] , DMF/NH 4 + [24] , [25] , [26] , etc). These reactions proceed through Rosenmund-von Braun reaction mechanism and suffer from limited catalytic efficiency and/or substrate scope due to strong coordination ability and poisoning of cyanide ion. Fig. 1: Catalytic cyanations with different cyano sources. a The use of metal cyanides, b organic cyano compounds, and c CO 2 /NH 3 as the CN source. Full size image Meanwhile, elegant development of cyanide-free methods involving diverse mechanisms to circumvent this challenge has been achieved including β-H elimination-facilitated cyanation [27] , [28] , electrophilic cyanation with N -cyano- N -phenyl- p -methylbenzenesulfonamide [29] , oxidative cyanation with tert -butyl isocyanide [30] , [31] or hexamethylenetetramine [32] etc. Besides, the recently emerging cyanation under reductive conditions as well undergoes different mechanisms, and in principle offers a complementary synthesis protocol for nitriles. Pioneering work by Cheng and co-workers used Pd/Ni-phosphine complexes for the catalytic cyanation of aryl halides with acetonitrile in the presence of zinc powder at 160 °C [33] . Also using Zn as reductant, Rousseaux and co-workers applied electrophilic cyanating reagent 2-methyl-2-phenyl malononitrile for the cyanation of aryl halides [34] . Very recently, Tsurugi and Mashima et al. developed the use of acetonitrile as cyano source using N -silylated dihydropyrazines as reductant [35] . However, to the best of our knowledge none of these systems are suitable for general cyanation of the least expensive and most widely available organic chlorides having the relatively inert C(sp 2 )-Cl bond (ca. 96 kcal mol −1 ). Therefore, there is an increasing need to develop general methods for cyanide-free cyanation of organic chlorides. In order to synthesize nitriles through reductive cyanation pathway, the use of higher oxidation state CO 2 as the carbon source is ideal for charge balance purpose. Accordingly, there are challenges to be overcome: (1) suppressing reductive dehalogenation; (2) suppressing the undesired CO 2 reduction; 3) conquering possible formation of stable urea, and (4) generation of active electrophile ready for C–C bond formation and C–N triple bond construction (Fig. 2 ). Accordingly, the choice of metal precursors and ligands is crucial to suppress the above mentioned side-reactions. Fig. 2: Challenges for reductive cyanation strategy. a Reductive dehalogenation. b reduction of CO 2 . c The generation of stable urea. d The challenging generation of active electrophiles. Full size image The discovery of cyanation reagents with operational simplicity and economic viability is a sought-after goal in organic synthesis. In this respect, CN source from sustainable C1 and N1 feedstocks is a natural line of enquiries. The fixation and transformation of carbon dioxide (CO 2 ) has attracted considerable attention [36] , [37] , [38] , [39] , [40] . Carbon dioxide is the most abundant carbon source, and is thus regarded as the most promising nontoxic C1 feedstock [41] , [42] , [43] , [44] , [45] , [46] . Recently, we developed the Cu-catalyzed reductive cyanation of aryl iodides with CO 2 /NH 3 as cyano (CN) source [47] . Herein, we report the reductive cyanation of organic chlorides using CO 2 /NH 3 or urea as either gaseous or solid forms of carbon and nitrogen, respectively (Fig. 1c ). 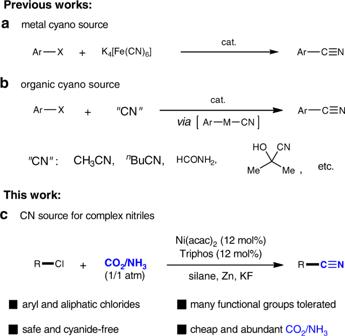Fig. 1: Catalytic cyanations with different cyano sources. aThe use of metal cyanides,borganic cyano compounds, andcCO2/NH3as the CN source. Reaction discovery Our study began by investigating catalytic cyanation of chlorobenzene with ambient CO 2 and NH 3 in the presence of PhSiH 3 and KF (Table 1 ). The model reaction was firstly tested with different metal catalysts (also see Supplementary Table 1 ). Among a wide range of catalysts examined, only nickel salts provided the desired product (Table 1 , entries 1–5). Further reaction optimization indicated that Ni(acac) 2 was a superior choice (entry 6). The addition of Zn powder as co-reductant promoted the reaction significantly raising the yield to 37% (Table 1 , entry 7). Gratifyingly, evaluation of ligands showed remarkable performance of Triphos for this transformation to produce 2a in 81% yield (Table 1 , entries 8–13). Screening of solvents and silane reductants were carried out. Other high boiling point polar solvents like DMI were found less suitable (Table 1 , entry 14). Notably, the choice of silanes also appeared to be crucial for the reaction with PMHS giving poor reactivity (Table 1 , entry 15). Table 1 Optimization of the reaction conditions a . Full size table Cyanation using CO 2 /NH 3 and the synthetic application Encouraged by the results above, we then investigated the utility and scope of this method. An array of aryl chlorides bearing various substituents were well-tolerated to afford the desired nitrile products in moderate to high yields (Fig. 3 ). 13 C-labeled benzonitrile 13 C- 2a was conveniently obtained using 13 CO 2 (83% yield), which confirmed that the carbon source of cyano moiety was derived from CO 2 (see Supplementary Figs 2 , 3 ). We found that substrates substituted with both electron-donating groups (alkyl, OMe, NH 2 , or OPh) as well as electron-withdrawing groups (F, CF 3 , CO 2 Me, or m -NHMe) underwent the cyanation reaction smoothly. Low yield ( 2o , 37%) was obtained for the reaction of 3-chlorobenzonitrile, with benzonitrile generated as the main by-product from dehalogenative hydrogenolysis. Aryl chlorides containing two substitutents at different positions were also readily cyanated ( 2p-2s , 69–92%). It is noteworthy that various reducible functional groups such as imine, ester, amide, and olefin groups were tolerated in this system [48] , [49] , [50] . 1,2-Diaryl olefin and trisubstituted olefin were found compatible giving products with acceptable yields ( 2x-2y , 36–93%). In contrast, C=C bond of 1,1-diarylethene 1z was reduced to give the product 2z (55% yield). We next proceeded to assess the applicability of this method in modifying bioactive intermediates ( 2aa-2ae ). And this method proved to be efficient in these cases with satisfactory yields obtained (57–94%). Specifically, cyanation of 2-chlorophenothiazine provided Cyamemazine precursor 2aa in excellent yield (94%). Lipid lowering agent Clofibrate was successfully cyanated to produce 2ab in modest yield (57%). Delightedly, cyanated products 2ac and 2ad were also obtained in 80% and 71% yields, respectively. In addition, transforming the anti-histaminic and anti-allergic Loratadine to nitrile 2ae was achieved in decent yield (72%). Furthermore, compounds 2ad , 2ae , 2ad’ , and 2ae’ were evaluated for their antiproliferative activity against MCF-7 and Hela cells. 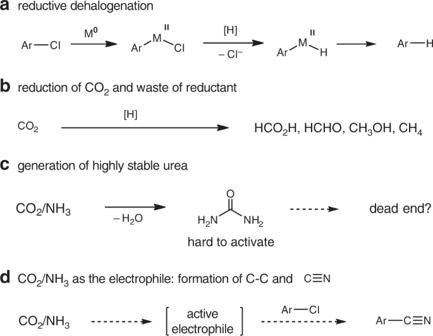Fig. 2: Challenges for reductive cyanation strategy. aReductive dehalogenation.breduction of CO2.cThe generation of stable urea.dThe challenging generation of active electrophiles. As shown in Fig. 4 , compounds 2ad and 2ae showed moderate antiproliferative activities against these cell lines with IC 50 values ranging from 5.91 to 23.54 μM, while compounds 2ad’ and 2ae’ showed no activities toward tumor cell lines MCF-7 and Hela with IC 50 > 50 μM. Fig. 3: Applicability study using CO 2 /NH 3 . Reaction conditions: 1 (0.125 mmol), CO 2 /NH 3 (1/1 atm), NMP (0.5 mL), 20 h, GC yield. a 13 CO 2 was used. b Isolated yields. c 15 mol% Ni(acac) 2 , 15 mol% Triphos. d 10 mol% Ni(acac) 2 , 10 mol% Triphos. Full size image Fig. 4: In vitro antiproliferative activities of compounds 2ad , 2ae , 2ad’ , and 2ae’ . a Concentration that inhibits the proliferation of cancer cells by 50%. Cell proliferation was measured using the CCK8 assay after incubation with the compounds for 24 h. The mean values of three independent experiments ± SE are reported. Full size image Cyanation with other CO 2 -derived CN sources Considering the easy access of many CO 2 -derived compounds, we tested our reductive cyanation approach using other types of CN sources (Fig. 5 ). The results showed that the presence of NH 2 moiety is crucial for the cyanation reactivity. To our delight, excellent yield could be obtained under the optimized conditions with urea (97% yield). Here, it is interesting to stress that silyl isocyanate TMS-NCO is an appropriate CN source giving 74% yield of the desired product. The involvement of isocyanate intermediates has already been established in our previous work on the use of CO 2 /NH 3 as the cyanating reagent [47] . Fig. 5: Catalytic cyanation with other related CN sources. Reaction conditions: 0.3 mmol scale; GC yields. a 2 equiv. of PhSiH 3 . Full size image Substrate scope using urea as CN source Since urea is a product of dehydration of ammonia and carbon dioxide, we then considered to evaluate urea as the cyano source for substrate scope screening. As shown from Fig. 6 , various functional groups were tolerated to producing the desired nitriles with excellent chemo-selectivity. Generally, substrates with electron rich group in the para -position showed higher reactivity ( 2e-2f , 2af-2ag ). Lowering reaction temperature, the transformation proceeded similarly with substrates bearing electron deficient substituents affording acceptable yields ( 2h-2i , 2k , 61–87%). Moreover, functional groups including hydroxyl, amino, methylamino, etc. at various positions on the aromatic ring remained unaltered even in the presence of excess reductant ( 2l-2m , 2ai-2ak ). The reactions proceeded smoothly for di-substituted substrates bearing methyl, alkoxy, amino, and trifluoromethyl groups ( 2q-2s , 2al-2am ). Various polycyclic aromatic skeletons, like naphthalene, indole, thianaphthene, and carbazole were also compatible, providing aromatic nitriles in moderate to excellent yield ( 2t-2v , 2an-2ax , 54–97%). 13 C-labeled nitrile compound was conveniently prepared in good yield using 13 C-urea ( 13 C- 2ax , 75%), and the product was characterized by NMR, HRMS, and single-crystal X-ray diffraction. Furthermore, heterocyclic substrates such as pyridine also showed gentle reactivity at 90 °C under optimized conditions. Direct reactions of chlorpromazine hydrochloride with urea delivered the corresponding product 2az in modest yield with promazine as side product due to dehalogenation. To our delight, metoclopramide was transformed into target product in moderate yield despite the multiple substituents ( 2ba , 76%). Notably, the system was suitable for benzyl chlorides when dppp ligand was used instead of Triphos, leading to the corresponding benzyl nitriles 2bb-2bf within a relatively short period of time (5 h; 35–85% yields). When cyclohexyl chloride or phenylethyl chloride were used as the substrate, desired products were also obtained, albeit in low yields (15–32%). Fig. 6: Substrate scope using urea. Reaction conditions: 1 (0.3 mmol), urea (3 equiv. ), NMP (1.0 mL), 20 h; GC yield. a Isolated yields. b 15 mol% Ni(acac) 2 , 15 mol% Triphos. c K 3 PO 4 was used instead of KF. d 13 C-urea was used. e From chlorpromazine hydrochloride, 1.5 equiv. KF. f dppp was used instead of Triphos. Full size image Mechanistic studies In order to examine the reactive species, we questioned whether the catalytic cyanation proceeded via an in situ generation of CN - . When tested with TMS-CN as cyanogen under standard conditions, cyanated product was undetected while substrate chlorobenzene was mostly recovered. This result suggests that CN - is not involved in the reaction. In addition, when Et 3 SiH was used as reductant, certain amounts of triethylsilyl isocyanate were detected even though cyanation product was not observed (Supplementary Fig. 4 ). Considering the thermolysis of urea to release isocyanic acid and ammonia, the formation of active silyl isocyanate intermediates is possible [51] , which is consistent with the results using TMS-NCO as shown in Fig. 5 . To further gather information on the active Ar–Ni species, several Ar–Ni complexes were prepared and used in stoichiometric reactions (Fig. 7 ). In these stoichiometric reactions, to avoid the possible unwanted F–Si interaction between KF and TMS-NCO, KF was added prior to TMS-NCO. First, product o -tolunitrile 2 o -Me was prepared from Ni( o -tolyl)(dppp), which was formed by transmetallation of (dppp) 2 Ni(BF 4 ) with o -tolylmagnesium chloride and TMS-NCO (Fig. 7a ). (Low yield of 6% for 2 o -Me is reasonable since o -chlorotoluene goes with dppp at standard conditions furnishing 2 o -Me in 11% yield.) Fig. 7: Stoichiometric reactions relevant to mechanism. a Reactivity of Ar–Ni(I) generated in situ. b Reactivity of Ar–Ni(II) generated in situ. c Reactivity of Ar–Ni(II). d Reactivity of Ar–Ni(III) generated in situ. Full size image These results revealed that Ni(I) species play an important role in the catalytic cycle [52] , [53] , [54] , [55] , [56] . Exposure of PhNi(dppp)Cl prepared by oxidative addition of 1a to Ni(dppp) 2 , with TMS-NCO failed to afford product 2a whereas 2a was obtained in 53% yield in the presence of PhSiH 3 (Fig. 7b ). Such experiment suggests that Ni(I) species are responsible for the reactivity while Ni(II) species are not critical for the reaction. Direct reaction of o -tolylNi(dppf)Cl and TMS-NCO did not produce the desired product 2 o -Me (only 2% yield when adding PhSiH 3 ), thus supporting that Ni(I) aromatic species are possible key intermediates (Fig. 7c ). Finally, the results of Ar–Ni(III) species generated in situ with TMS-NCO are in line with the pathway that Ni(I) species react with silyl isocyanates to form the C–C bond (Fig. 7d ). Based on these experimental results and previous reports [57] , [58] , [59] , a possible reaction pathway is proposed as shown in Fig. 8 . First, Ni(II)-precursors are reduced to Ni(0)-species A in the presence of silanes and Zn. This is followed by oxidative addition of the aryl chloride to A to form Ni(II) halide B , which is reduced by silane and Zn to afford highly nucleophilic Ni(I) intermediate C . Subsequently, silyl isocyanates formation [51] is followed by nickel–carbon insertion to generate presumably transient imidate species D . Further transformation yields the cyano product via a plausible 1,3-silyl N-to-O migration, whereby nickel siliconate intermediate E is released and further reduced by hydrosilane to regenerate species A . As discussed before, the formation of aryl-Ni(I) species is critical, while species C is stabilized by the tridentate phosphine ligand Triphos. The other advantage using Triphos is that it can act as the bidentate ligand favoring the formation of species B and D via addition reactions. The presence of Zn retarded the dehalogenative reduction process probably via inhibiting the formation of Ni(II)-hydride species [60] . The addition of alkali metal chlorides such as LiCl can promote the reduction of Ni(II) complex to Ni(0) species by zinc flakes [61] and accordingly the addition of KF is likely to promote the reduction of Ni(II) species B to Ni(I) species C . In summary, we have demonstrated the catalytic reductive cyanation of nonactivated aryl/heteroaryl and aliphatic chlorides with CO 2 /NH 3 as cyano source. In the presence of nickel–triphos complexes, various organic chlorides were transformed into the desired aryl nitriles in moderate to excellent yields (up to 97%). Remarkably, diverse functional groups including nucleophilic hydroxyl, amino, unsaturated ester, amide, and olefin and heterocycle groups were tolerated. Cheap and bench-stable urea is also a proper CN source in this catalytic system, making it attractive to applications. Mechanistic studies demonstrate that Ar–Ni(I) species are responsible for the C–C coupling through the active silyl isocyanate intermediates. 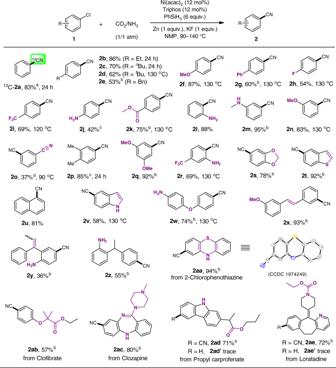Fig. 3: Applicability study using CO2/NH3. Reaction conditions:1(0.125 mmol), CO2/NH3(1/1 atm), NMP (0.5 mL), 20 h, GC yield.a 13CO2was used.bIsolated yields.c15 mol% Ni(acac)2, 15 mol% Triphos.d10 mol% Ni(acac)2, 10 mol% Triphos. Fig. 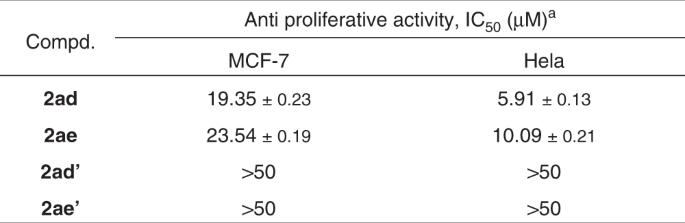Fig. 4: In vitro antiproliferative activities of compounds2ad,2ae,2ad’, and2ae’. aConcentration that inhibits the proliferation of cancer cells by 50%. Cell proliferation was measured using the CCK8 assay after incubation with the compounds for 24 h. The mean values of three independent experiments ± SE are reported. 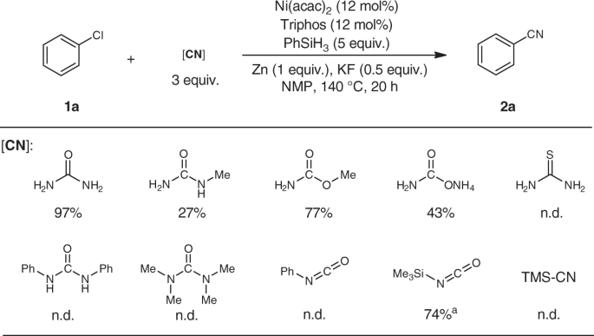Fig. 5: Catalytic cyanation with other related CN sources. Reaction conditions: 0.3 mmol scale; GC yields.a2 equiv. of PhSiH3. 8: Plausible reaction mechanism. 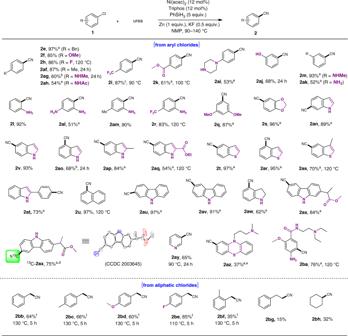Fig. 6: Substrate scope using urea. Reaction conditions:1(0.3 mmol), urea (3 equiv.), NMP (1.0 mL), 20 h; GC yield.aIsolated yields.b15 mol% Ni(acac)2, 15 mol% Triphos.cK3PO4was used instead of KF.d 13C-urea was used.eFrom chlorpromazine hydrochloride, 1.5 equiv. KF.fdppp was used instead of Triphos. Ni/phosphine-catalyzed reductive cyanation of organic chlorides using CO 2 /NH 3 . Full size image 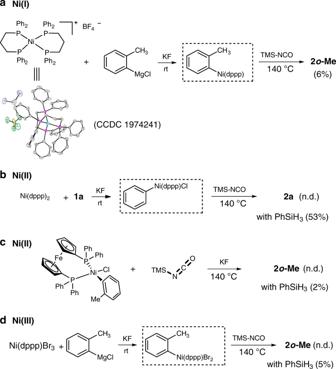Fig. 7: Stoichiometric reactions relevant to mechanism. aReactivity of Ar–Ni(I) generated in situ.bReactivity of Ar–Ni(II) generated in situ.cReactivity of Ar–Ni(II).dReactivity of Ar–Ni(III) generated in situ. 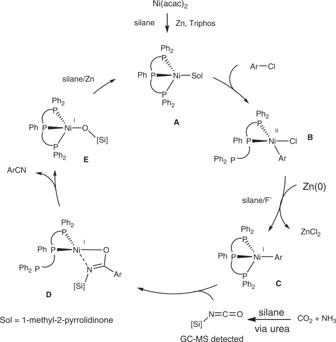Fig. 8: Plausible reaction mechanism. Ni/phosphine-catalyzed reductive cyanation of organic chlorides using CO2/NH3. General procedure for catalytic cyanation using CO 2 /NH 3 Under nitrogen atmosphere, Ni(acac) 2 (12 mol%, 0.015 mmol), Triphos (12 mol%, 0.015 mmol), KF (1.0 equiv., 0.125 mmol), Zn (1.0 equiv., 0.125 mmol), and a stirring bar were added into a 10 mL oven-dried sealed tube. Then NMP (0.5 mL), aryl chlorides (1.0 equiv., 0.125 mmol), and PhSiH 3 (6.0 equiv., 0.75 mmol) were injected by syringe. The tube was sealed and CO 2 (3.6 equiv., 10 mL) as well as NH 3 (3.6 equiv., 10 mL) were injected by syringe after N 2 was removed under vacuum. Then the mixture was stirred for 20 h in a preheated alloyed block. After the reaction finished, the tube was cooled to room temperature and the pressure was carefully released. The yield was measured by GC analysis or isolated by preparative thin-layer chromatography on silica gel plates eluting with PE/EtOAc.